Motional averaging in a superconducting qubit Superconducting circuits with Josephson junctions are promising candidates for developing future quantum technologies. Of particular interest is to use these circuits to study effects that typically occur in complex condensed-matter systems. Here we employ a superconducting quantum bit—a transmon—to perform an analogue simulation of motional averaging, a phenomenon initially observed in nuclear magnetic resonance spectroscopy. By modulating the flux bias of a transmon with controllable pseudo-random telegraph noise we create a stochastic jump of its energy level separation between two discrete values. When the jumping is faster than a dynamical threshold set by the frequency displacement of the levels, the initially separate spectral lines merge into a single, narrow, motional-averaged line. With sinusoidal modulation a complex pattern of additional sidebands is observed. We show that the modulated system remains quantum coherent, with modified transition frequencies, Rabi couplings, and dephasing rates. These results represent the first steps towards more advanced quantum simulations using artificial atoms. The ability to resolve energy variations Δ E occurring in a time interval Δ t is fundamentally limited by the energy-time uncertainty relation . Consider for example a system of spin-1/2 particles filling a porous material ( Fig. 1a ) in an external magnetic field; then, if the pore wall is paramagnetic, the particles near it will experience a modified local magnetic field. As a result, static particles will produce two spectral peaks in the nuclear magnetic resonance spectrum at frequencies ω 1 and ω 2 ( Fig. 1b ). In contrast, particles moving swiftly back and forth between the two regions on timescales Δ t shorter than are not able to discriminate between the two energy values. Then, as the particles move faster, the outcome in the spectroscopy is not simply a continuous broadening and overlapping of the two peaks. Instead, a new peak emerges at the average frequency ω 0 with a width smaller than the energy separation , denoted as motional averaging and narrowing [1] , [2] , respectively. In atomic ensembles and condensed-matter systems, this occurs via fast variations of the electronic state populations, chemical potential, molecular conformation, effective magnetic fields, lattice vibrations, micro-electric fields producing ac-Stark shifts and so on [1] , [2] , [3] , [4] , [5] , [6] . Closely related phenomena are the Dyakonov-Perel effect [7] , the Dicke line narrowing of Doppler spectra [8] , and the quantum Zeno effect [9] . 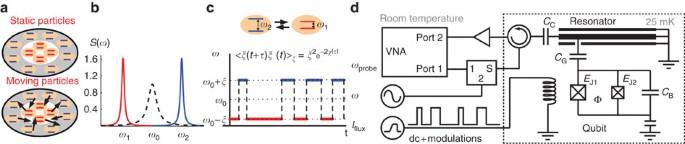Figure 1: Schematics of motional averaging and simplified experimental set-up. (a) Illustration of a single pore filled with a medium consisting of spin-1/2 particles that are either static or moving. White and grey areas denote different magnetic environments, producing the energy splittingsand, respectively (seeb,c). (b) Schematic spectrum of the motional averaging. The solid lines denote the spectrum of static particles, while the dashed line corresponds to moving particles. (c) A sample trajectory of the energy splittingin equation (1). (d) Schematic diagram of the sample device and the simplified experimental set-up. Two asymmetric Josephson junctions (EJ1andEJ2) are capacitively shunted (CB) and coupled (CG) to a resonator. The time-dependent transition frequency of the qubit is controlled with fast flux pulses on top of a dc bias (Iflux=Idc+Ipulse), generated by an AWG. A vector network analyser (VNA) is used for probing the resonator atωprobe≈ωr. One microwave source (ω) is used for driving the qubit. Additional details are shown in Methods and inSupplementary Fig. S1. Figure 1: Schematics of motional averaging and simplified experimental set-up. ( a ) Illustration of a single pore filled with a medium consisting of spin-1/2 particles that are either static or moving. White and grey areas denote different magnetic environments, producing the energy splittings and , respectively (see b , c ). ( b ) Schematic spectrum of the motional averaging. The solid lines denote the spectrum of static particles, while the dashed line corresponds to moving particles. ( c ) A sample trajectory of the energy splitting in equation (1). ( d ) Schematic diagram of the sample device and the simplified experimental set-up. Two asymmetric Josephson junctions ( E J1 and E J2 ) are capacitively shunted ( C B ) and coupled ( C G ) to a resonator. The time-dependent transition frequency of the qubit is controlled with fast flux pulses on top of a dc bias ( I flux = I dc + I pulse ), generated by an AWG. A vector network analyser (VNA) is used for probing the resonator at ω probe ≈ ω r . One microwave source ( ω ) is used for driving the qubit. Additional details are shown in Methods and in Supplementary Fig. S1 . Full size image In this paper, we report the observation of motional averaging and narrowing in a single artificial atom, a quantum bit (qubit), with a simulated fast-fluctuating environment under direct experimental control. This should be contrasted with the typical situation in condensed-matter systems, where one has a large number of particles and the experimentalist can only indirectly attempt to change the fluctuation rate, typically by modifying a thermodynamic function of state, such as temperature or pressure. Frequency-modulated transmon qubit Our device is a circuit QED system [10] , consisting of a tunable transmon coupled to a quarter-wavelength coplanar waveguide resonator. The circuit schematic and the simplified experimental set-up are shown in Fig. 1d and in Supplementary Fig. S1 . The applied bias flux Φ through the qubit loop consists of a constant part Φ dc and a time-dependent part Φ ac ( t ) with an amplitude much smaller than Φ dc . The Hamiltonian of the transmon qubit [11] is where . Here Φ 0 = h /2 e is the magnetic flux quantum, the Josephson plasma frequency is , denote the Pauli matrices, the single-electron charging energy is E C = e 2 /2( C G + C B )≈ h × 0.35 GHz, E J = E J1 + E J2 ≈24 E C is the maximum Josephson energy, and d =( E J1 − E J2 )/ E J ≈0.11 denotes the junction asymmetry. We choose Φ dc so that ω 0 /2 π =2.62 GHz, which is far detuned from the bare resonator frequency ω r /2 π =3.795 GHz, allowing the dispersive measurement of the qubit through the resonator by standard homodyne and heterodyne techniques [12] . The time-dependent part of the energy splitting, determined by Φ ac ( t ), is controlled by an arbitrary waveform generator (AWG) via a fast flux line. The random telegraph noise (RTN) is realized by feeding pseudo-random rectangular pulses to the on-chip flux bias coil. Ideally, the dynamics of is a stationary, dichotomous Markovian process, characterized by an average jumping rate χ and symmetrical dwellings at frequency values of ± ξ (see Fig. 1c ). The number of jumps is a Poisson process with the probability P n ( t )=( χt ) n e − χt / n ! for exactly n jumps within a time interval t . This Poissonian process simulates the temporal variations causing motional averaging in atomic ensembles and condensed-matter systems ( Fig. 1 ). Simulation of motional averaging In order to find the effective transition energies and decoherence rates of the modulated system, we calculate the absorption spectrum [1] , [2] . For a qubit subjected to RTN fluctuations as in equation (1), we exploit the quantum regression theorem [13] to find the spectrum (see details in Supplementary Note S1 ) where the expectation value is taken over noise realizations and Γ 2 = Γ ϕ + Γ 1 /2 is the decoherence rate in the absence of modulation. For our sample Γ 2 ≈2 π × 3 MHz (determined in an independent measurement). For the Poisson process ξ ( t ), equation (2) gives [1] , [2] , [14] , [15] with and . In our measurement, we have recorded the population of qubit's excited state, as shown in Fig. 2 and in Supplementary Fig. S2 . 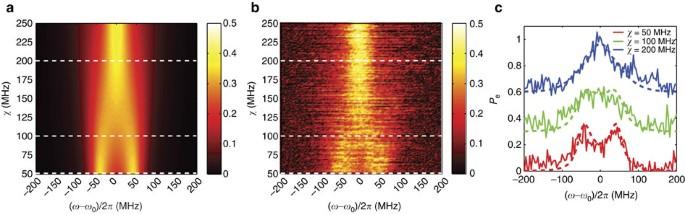Figure 2: Motional averaging. (a) Numerical simulation of the occupation probabilityPeplotted in theω−χplane with parametersξ/2π=43 MHz,g/2π=8 MHz,Γ1/2π=1 MHz, andΓ2/2π=3 MHz. (b) Measured excited state occupation probabilityPeunder the RTN modulation. (c) Horizontal cuts of the measured occupation probability inb, denoted with white lines, at three different jumping rates (solid lines). For clarity, the curves are displaced vertically by 0.3. The dashed lines indicate the corresponding results of the numerical simulation ina. SeeSupplementary Fig. S2for the zero-detuning (ω=ω0) occupation probabilityPewith differentξ. The qubit is excited with a transverse drive Figure 2: Motional averaging. ( a ) Numerical simulation of the occupation probability P e plotted in the ω − χ plane with parameters ξ /2 π =43 MHz, g /2 π =8 MHz, Γ 1 /2 π =1 MHz, and Γ 2 /2 π =3 MHz. ( b ) Measured excited state occupation probability P e under the RTN modulation. ( c ) Horizontal cuts of the measured occupation probability in b , denoted with white lines, at three different jumping rates (solid lines). For clarity, the curves are displaced vertically by 0.3. The dashed lines indicate the corresponding results of the numerical simulation in a . See Supplementary Fig. S2 for the zero-detuning ( ω = ω 0 ) occupation probability P e with different ξ . Full size image The simulation of the occupation probability presented in Fig. 2a (see Methods and Supplementary Note S2 ) includes also the effect of power broadening due to strong driving amplitudes ( g > Γ 1 , Γ 2 ). Two intuitively appealing limits result from equation (3) (see also Fig. 2 ) at the opposite sides of a dynamical threshold defined by χ = ξ . In the case of slow jumping, , and resolvable energy variations, , the qubit absorbs energy at ω 0 ± ξ with the total decoherence rate . The correlation time of the displacement process is τ ξ =(2 χ ) −1 and the linewidth (full width at half maximum ) broadens by the amount of the reduced mean life-time of a qubit excitation (exchange broadening [1] ). In contrast, for fast jumping processes, , and when the variations are not resolvable, , the qubit absorbs energy only at the frequency ω 0 with . The increase in decoherence rate by ξ 2 /2 χ can be related to the excursions of the accumulated phase (equation (2)) for single noise realizations, especially to the diffusion coefficient of the process [16] . Surprisingly, the averaged spectral line is well-localized around the mean value, since . The effect of motional narrowing can be best seen in Fig. 2c as a raise in the height of the centre peak because the additional decoherence ξ 2 /2 χ decreases with increasing jumping rate χ . When χ is comparable with ξ , there is a cross-over region where absorption is reduced and the peak broadens due to enhanced decoherence (see Fig. 2 ). This is important for the improvement of qubit dephasing times as it implies that a longitudinally coupled two-level system (TLS) fluctuator is the most poisonous when its internal dynamics occurs approximately at the same frequency as the coupling to the qubit. A counter-intuitive aspect of motional averaging is that the system is at any time in either one of the states and spends no time in-between. Yet spectroscopically it is not seen in the states ; instead it has a clear signature in the middle. Also, the spectrum (3) decays as 1/ ω 4 far in the wings, showing a non-Lorentzian character that originates from the non-exponential decay of the correlator [14] . This is because the frequent -changes have a similar effect to a continuous measurement of the system, slowing its dynamics in analogy with the quantum Zeno effect [9] , [17] . Sinusoidal modulation of frequency To further explore these effects, we have used sinusoidal waves to modulate the qubit energy splitting: . In Fig. 3a , the experimental data and the corresponding numerical simulation are shown. Resolved sidebands appear at ω = ω 0 ± k Ω ( k =0,1,2,…), and are amplitude-modulated with Bessel functions J k ( δ /Ω), where δ and Ω denote the modulation amplitude and frequency, respectively. The Hamiltonian (equations (1) and (4)) can be transformed to a non-uniformly rotating frame [18] , [19] (see Methods). 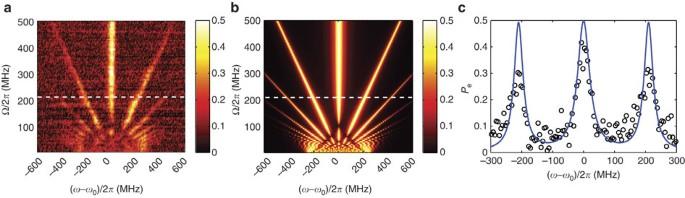Figure 3: Occupation probabilities of the excited state of the qubit under sinusoidal modulations. (a) Measured excited state occupation probabilityPewith amplitudeδ/2π=250 MHz. (b) Simulation withΓ1/2π=1 MHz,Γ2/2π=3 MHz, andg/2π=20 MHz.cThe cut along the dashed line ina,bat Ω/2π=210 MHz. The (black) circles are the experimental data. The (blue) line denotes the analytical occupation probability obtained from equation (5) by takingk=−1,0,1, which overlaps perfectly with the simulation in the parameter regime,. Fork=0 (0-band), the linewidth is narrower than the bare linewidth without modulation (see Methods andSupplementary Fig. S3). The theoretical prediction for the steady-state occupation probability on the resolved sidebands (Ω> g > Γ 2 ) is Figure 3: Occupation probabilities of the excited state of the qubit under sinusoidal modulations. ( a ) Measured excited state occupation probability P e with amplitude δ /2 π =250 MHz. ( b ) Simulation with Γ 1 /2 π =1 MHz, Γ 2 /2 π =3 MHz, and g /2 π =20 MHz. c The cut along the dashed line in a , b at Ω/2 π =210 MHz. The (black) circles are the experimental data. The (blue) line denotes the analytical occupation probability obtained from equation (5) by taking k =−1,0,1, which overlaps perfectly with the simulation in the parameter regime, . For k =0 (0-band), the linewidth is narrower than the bare linewidth without modulation (see Methods and Supplementary Fig. S3 ). Full size image which is compared with experimental data in Fig. 3c and in Supplementary Fig. S3 . These population oscillations can be alternatively understood as a photon-assisted version of the standard Landau–Zener–Stückelberg interference [20] , [21] (see Methods and Supplementary Fig. S4 ). Also, when the qubit drive is tuned close to the resonator frequency ω ≈ ω r and when the driving amplitude g is large and equal to the frequency of the modulation g =Ω, the system can be seen as a realization of a quantum simulator of the ultrastrong coupling regime [22] , [23] . In our set-up, the simulated coupling rate is estimated to reach over 10% of the effective resonator frequency (see Supplementary Note S3 ), comparable to earlier reports [24] , [25] where the ultrastrong coupling was obtained by sample design. The sinusoidal modulation allows a different perspective on motional averaging. The RTN noise comprises many different modulation frequencies Ω ( Fig. 1c ). Each frequency creates different sidebands ( k =1,2,3,…), which overlap and average away. At large Ω's only the central band k =0 survives because the only non-vanishing Bessel function of zero argument is J 0 (0)=1. Coherence of the modulated system Finally, we show that it is possible to use the modulated system as a new, photon-dressed qubit. Indeed, we can drive Rabi oscillations on the central band and on the resolved sidebands (see Fig. 4 and Supplementary Fig. S5 ). For fast RTN modulation, , and under the strong drive in equation (4), we construct (see Supplementary Note S2 ) a master equation [15] describing the Rabi-oscillation with the detuned Rabi frequency and with the total decoherence rate . In the case of sinusoidal modulation, the Rabi frequencies on the sidebands are obtained as . 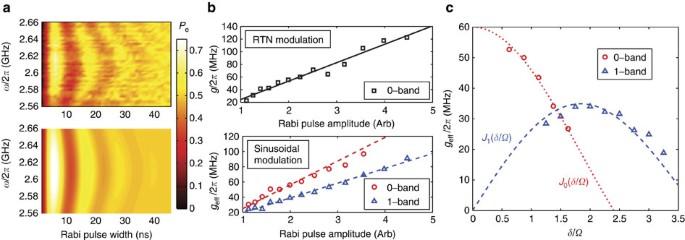Figure 4: Rabi oscillations with modulations. (a) Rabi oscillations versus driving frequency with RTN modulation: measurement and numerical simulation withω0/2π=2.610 GHz,ξ/2π≈95 MHz,χ≈600 MHz,g/2π=91 MHz,Γ1/2π=1 MHz, andΓ2/2π=3 MHz. The corresponding Rabi oscillations in the case of sinusoidal modulation are shown inSupplementary Fig. S5. (b) The measured Rabi frequency of the random and sinusoidal modulationgandgeff, respectively, as a function of Rabi-pulse amplitude (same scaling in the both panels). The solid and dashed lines are fits to the data in the linear regime. (c) Rabi frequencies versus amplitude of the sinusoidal modulation. The horizontal axis is the dimensionless scaled modulation amplitudeδ/Ω, which is also the argument for the effective Rabi frequencyplotted withg/2π=60 MHz and colour coding fork: 0 (red dotted) and 1 (blue dashed). The (red) circles and (blue) triangles indicate the measured Rabi frequencies at the centre of 0-band and 1-band, respectively. Figure 4: Rabi oscillations with modulations. ( a ) Rabi oscillations versus driving frequency with RTN modulation: measurement and numerical simulation with ω 0 /2 π =2.610 GHz, ξ /2 π ≈95 MHz, χ ≈600 MHz, g /2 π =91 MHz, Γ 1 /2 π =1 MHz, and Γ 2 /2 π =3 MHz. The corresponding Rabi oscillations in the case of sinusoidal modulation are shown in Supplementary Fig. S5 . ( b ) The measured Rabi frequency of the random and sinusoidal modulation g and g eff , respectively, as a function of Rabi-pulse amplitude (same scaling in the both panels). The solid and dashed lines are fits to the data in the linear regime. ( c ) Rabi frequencies versus amplitude of the sinusoidal modulation. The horizontal axis is the dimensionless scaled modulation amplitude δ /Ω, which is also the argument for the effective Rabi frequency plotted with g /2 π =60 MHz and colour coding for k : 0 (red dotted) and 1 (blue dashed). The (red) circles and (blue) triangles indicate the measured Rabi frequencies at the centre of 0-band and 1-band, respectively. Full size image Our work could open up several research directions. For example, a key limitation in solid-state based quantum processing of information is the decoherence due to fluctuating TLSs in the dielectric layers fabricated on-chip [26] , [27] , [28] . We anticipate, resting on the motional narrowing phenomenon, that the dephasing times of the existing superconducting qubits may be dramatically improved if one is able to accelerate the dynamics of the longitudinally coupled TLSs. The quantum coherence of the resolved sidebands and of the central band suggest that low-frequency modulation offers an additional tool for implementing quantum gates [29] , in analogy with the use of vibrational sidebands in the ion trap computers [30] . Also, if the two tones used to drive and modulate the qubit satisfy certain conditions, the system can be mapped into an effective qubit-harmonic oscillator system with ultrastrong coupling, opening this regime for experimental investigations. Finally, the recent progress in the field of nanomechanical oscillators makes possible the study of frequency jumps in nanomechanical resonators [16] , which is predicted to be accompanied by squeezing [31] . Our work paves the way for further simulations of quantum coherence phenomena using superconducting quantum circuits [32] , [33] . Measurement set-up The electronic measurement set-up at room temperature is illustrated in Supplementary Fig. S1 . For qubit spectroscopy with RTN modulations, the dc flux bias and RTN modulations are generated by an Agilent 81150A AWG. The qubit driving signal from an Agilent E8257D analogue signal generator and the coplanar waveguide cavity probe signal from an Agilent N5230C PNA-L network analyser are combined together by a Mini-Circuits ZFSC-2-10G power splitter/combiner and sent to the cavity input line of the dilution refrigerator. The signal from the cavity output line of the dilution refrigerator is amplified and detected by a PNA-L network analyser. For sinusoidal modulations, the tones are generated by a R&S SMR27 microwave signal generator and they are added to the dc bias generated by the Agilent 81150A via a bias tee (not shown). Between the radio frequency instruments (analogue signal generator and network analyser) and their corresponding lines, dc blocks are used for breaking possible ground loops. All instruments are synchronized with a SRS FS725 Rubidium frequency standard (not shown in the figure). For Rabi-oscillation measurements, high ON/OFF ratio Rabi pulses are generated by mixing a continuous microwave signal from the Agilent E8257D with rectangular pulses from a SRS DG645 digital delay generator via two identical Mini-Circuits frequency mixers. The Agilent N5230C PNA-L is used as a signal generator. Its output signal is split into two parts. One part is used for generating measurement pulses in a similar fashion to the Rabi pulses; the other part acts as a local oscillator signal to mix the output signal from the coplanar waveguide cavity down via a Marki IQ mixer. The IQ data is filtered, amplified by a SRS SR445A pre-amplifier, and digitized by an Agilent U1082A-001 digitiser. Measurement controlling and data processing are done by MATLAB running on a measurement computer. The communication between the measurement computer and the instruments is realized through IEEE-488 GPIB buses. To generate RTN pulses, we use MATLAB’s internal Poisson random number generator poissrnd( λ ) to obtain binary RTN sequences, and load the sequences into the Agilent 81150A AWG. Each binary RTN sequence consists of 50,000 data points and around 5,000 random jumps in average. The mean jumping rate χ (of AWG's output) is modulated by changing the clock frequency ν of the AWG: χ ≈5,000 × ν . To verify this relation between χ and ν , we observe the RTN sequences at different ν 's by a fast oscilloscope (10 GS per s), count the number n of edges (jumping events) for certain period of time t , and calculate the real mean jumping rate by its original definition, χ = n / t . As an example, a 0.5-μs long RTN sequence with estimated mean jumping rate χ ≈5,000 × 10 KHz=50 MHz is shown in Supplementary Fig. S1 . Twenty-five jumps are counted during 0.5 μs, which gives χ =50 MHz. As long as ν <100 KHz, the formula χ ≈5,000 × ν gives a good estimation of the mean jumping rate. For ν >100 KHz, the real mean jumping rate is smaller than the estimated one, due to the intrinsic ∼ 2 ns rising/falling time of the AWG. Numerical simulations The occupation probability of Figs 2a , c , 3b , and Supplementary Figs S2 and S4 is a result of solving numerically the master equation in the frame rotating at ω and applying the rotating wave approximation (the pure dephasing rate Γ ϕ = Γ 2 − Γ 1 /2). For the random modulation ( Figs 2a , c , and Supplementary Fig. S2 ), we apply the method of quantum trajectories [13] and the imperfections of the experimentally realized wave forms (the raising/falling time ∼ 2.0 ns and the sampling time 0.5 ns) are included in the simulation. Multi-photon transition process in sinusoidal modulation The effects of sinusoidally modulating the transition frequency of an atom is a generic problem in theoretical physics, and has attracted a lot of interest in the past, most notably in the quantum-optics community [34] , [35] . We address now this problem in the context of superconducting qubits. We consider a transmon qubit whose energy splitting is modulated sinusoidally: . Even though , the qubit can be excited with the low-frequency signal in the presence of an additional high-frequency drive ω . This can be seen as a multi-photon transition process involving quanta from both fields (in equation (5)), or, as a photon-assisted Landau–Zener–Stückelberg (LZS) interference [18] , [20] , [21] , [36] between the dressed states |↓, n 〉 and |↑, n −1〉. Let us first consider the multi-photon transition processes associated with the sinusoidal-modulated Hamiltonian, defined in equations (1) and (4), The qubit is driven both in the longitudinal ( ) and in the transverse ( ) direction. We show below how to eliminate the time-dependence from the longitudinal drive. After moving to a non-uniformly rotating frame with the unitary transformation [18] , [19] the effective Hamiltonian is , and by using the Jacobi-Anger relations, we get By assuming that the transverse drive is close to a resonance, that is, ω ≈ ω 0 ± k Ω ( k =0,1,2…) and that the resonances are resolvable Ω> g > Γ 2 , we transform back with and ignore all but the resonant terms, that is, all the fast rotating terms (rotating wave approximation, RWA). The resulting RWA Hamiltonian reads describing, in the Bloch spin representation, precessions around the vector Ω=( gJ k ( δ /Ω),0, ω 0 + k Ω− ω ) with the effective Rabi frequency Exactly at the multi-photon resonance ω = ω 0 ± k Ω ( k =0,1,2…), the effective Rabi frequency is | gJ k ( δ /Ω)|, and it is plotted in Fig. 4c . In the time domain, the measured Rabi oscillations are presented in Supplementary Fig. S5 together with numerical simulations of Bloch equations exploiting the effective Rabi frequency in equation (11). To find the steady-state occupation probability in the presence of relaxation with rate Γ 1 and decoherence with rate Γ 2 , we solve the Bloch equations analytically. In the RWA, that is when Ω> g > Γ 2 is satisfied, one is allowed to add up independent contributions from all the resonances (the resolved sidebands). The result for the steady-state excited state occupation probability is equation (5). In the non-modulated case, the corresponding expression for the occupations is simply The occupation probabilities in equations (5) and (12) are compared with the experimental steady-state occupation probabilities in Supplementary Fig. S3 . An interesting effect is that the linewidth of the modulated qubit on the central band is always smaller than the linewidth on the qubit in the absence of the modulation due to reduced power broadening. Photon-assisted Landau–Zener–Stückelberg interference The spectra seen in the experiment under sinusoidal modulation can be also interpreted as a photon-assisted LZS effect. Note that in the absence of the driving field standard LZS processes are not possible: indeed the qubit energy separation is one order of magnitude higher than the modulation frequency, therefore the standard LZS probability is negligibly small. However, the system can still perform LZS transitions by absorbing a photon from the driving field. This photon-assisted LZS interference can be seen by transforming the Hamiltonian from equation (7) into the frame rotating at ω around the z axis (unitary transformation ), where it has exactly the same form (in the RWA) as that of LZS interference [18] , [21] , [36] , namely As illustrated in Supplementary Fig. S4 , LZS transition events may occur when the modulation amplitude δ is of the order of, or larger than, the detuning between the driving frequency and the qubit splitting ω – ω 0 . The LZS transitions occur between the transversely dressed states |↓, n 〉 and |↑, n −1〉, where n refers to the photon number of the transverse driving field. The phase difference of the two states gathered between the consecutive tunnelling events leads to either constructive or destructive interference observed as maxima or minima in the occupation probability of the excited state, shown in Supplementary Fig. S4 . The LZS interference seen in our system corresponds to the so-called fast passage limit [21] . In this limit, the expression for the occupation probability can be calculated analytically [21] and the result agrees exactly with our equation (5). To prove experimentally that this picture is valid, we have scanned the modulation amplitude δ and the driving frequency ω at fixed Ω. We observe an interference pattern of the steady-state occupation probability, which is in good agreement with the theoretical prediction, see Supplementary Fig. S4 . How to cite this article: Li. J. et al. Motional averaging in a superconducting qubit. Nat. Commun. 4:1420 doi: 10.1038/ncomms2383 (2013).